Helium anomalies suggest a fluid pathway from mantle to trench during the 2011 Tohoku-Oki earthquake Geophysical evidence suggests that fluids along fault planes have an important role in generating earthquakes; however, the nature of these fluids has not been well defined. The 2011 magnitude 9.0 Tohoku-Oki earthquake ruptured the interface between the subducting Pacific plate and the overlying Okhotsk plate. Here we report a sharp increase in mantle-derived helium in bottom seawater near the rupture zone 1 month after the earthquake. The timing and location indicate that fluids were released from the mantle on the seafloor along the plate interface. The movement of the fluids was rapid, with a velocity of ~4 km per day and an uncertainty factor of four. This rate is much faster than what would be expected from pressure-gradient propagation, suggesting that over-pressurized fluid is discharged along the plate interface. Most great earthquakes occur at convergent plate boundaries in circum-Pacific regions [1] . Pore fluid along the interface between the descending oceanic plate and the over-riding plate might play an important role in the occurrence of these earthquakes [2] . This fluid increases the pore pressure, which may decrease the effective normal stress under a tectonic stress field, thereby triggering an earthquake [3] . The M9.0 Tohoku-Oki earthquake occurred at the plate interface between the Pacific plate and the Okhotsk plate [4] , [5] . The presence of elevated pore-fluid pressure in the megathrust zone is suggested by a temporal change in the stress field [6] and a landward increase in the wave amplitude of the seismic reflection properties [7] . A numerical simulation implies that the pore-fluid pressure distribution along the plate interface likely caused a shallow asperity of the earthquake [8] . Our study evaluates the geochemical nature and behaviour of pore-fluids along the interface between the two plates. Helium isotopes are useful in identifying the origin of fluids and may provide the key information about the source of interplate fluids. Here we show helium-3 anomalies in bottom seawater in the region near the Japan Trench after the M9.0 earthquake and suggest that the rupture of subduction plates may provide a pathway that connects the mantle wedge to the trench surface. This is the first evidence of a sudden emanation of mantle helium related to an interplate earthquake in the subduction zone, which may provide insight into the movement of mantle-derived fluids. Helium isotopes of bottom seawater We collected bottom seawater samples at four sites on the seafloor at depths from 1,779 to 5,699 m in the frontal arc region of NE Japan ~1 month after the M9.0 earthquake ( Fig. 1 , Methods). A second set of bottom seawater samples was taken at six sites on 16 June 2011. In addition, we collected deep-sea sediment and pore-water samples (Methods) at the coseismic slip region in August 2011, and their helium isotope compositions were measured in the laboratory. The observed excess of 3 He in the 15 samples from April was 16–20% ( Fig. 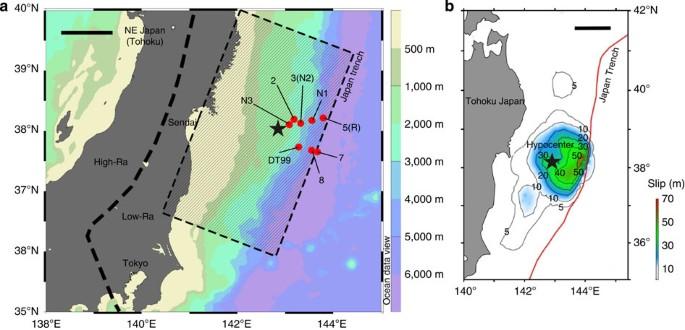Figure 1: Bottom seawater sampling sites in the Japan Trench. (a) Sampling sites of bottom seawater. The displaced fault plane is shown as a box with thin hatched lines4. The dashed line and star indicate the volcanic front and hypocenter, respectively. The black bar at the top left denotes a 100-km scale bar. (b) The size of the coseismic slip during the earthquake estimated by land and seafloor geodesy19. The black bar at the top right denotes a 100-km scale bar. 2 ; Supplementary Table 1 ), where excess 3 He is calculated as (Ra-1) × 100 and Ra is the observed 3 He/ 4 He ratio relative to the atmospheric ratio of 1.4 × 10 −6 (ref. 9 ). The northwest Pacific bottom seawater consistently shows elevated 3 He compared with atmospheric values: excess 3 He values of 18% at 2,000 m ( Supplementary Figs 1 and 2 ) result from abyssal currents dispersing mantle 3 He released from mid-oceanic-ridge volcanism [10] , which explains why the 3 He/ 4 He ratios decrease with increasing depth at sites N1 and N2 (grey shades in Fig. 2c,d ). The conditions were in a steady state before the earthquake, with similar 3 He/ 4 He values recorded since 2007, but the samples collected on April 15 showed equal or higher 3 He/ 4 He ratios than those before the earthquake (solid red circles in Fig. 2b–e ). An increase in 3 He is recorded at all sites after the M9.0 earthquake. Although the difference is small, the increase is statistically valid (Methods). The 3 He/ 4 He and 4 He/ 20 Ne ratios in the 16 June samples are similar to those from 15 April ( Supplementary Table 1 ). A detailed examination of the data indicates that the 3 He/ 4 He ratios in samples collected at shallower depths than 5,000 km (2-1, 3-1, DT99-5) are consistent with the pre-earthquake 3 He/ 4 He depth profile; however, those from deeper samples, >5,000 m, show more elevated ratios than the pre-earthquake profile ( Supplementary Fig. 3 ). 3 He/ 4 He ratios of deep-sea sediment and pore water samples in the trench region are 0.11–0.79 and 0.68–0.71 Ra, respectively ( Supplementary Tables 2 and 3 ). 4 He/ 20 Ne ratios are greater than the atmosphere value. The large variation in the 3 He/ 4 He of the solid sediments is explained by variation in the ratio of crustal material to the sediment (Methods). Figure 1: Bottom seawater sampling sites in the Japan Trench. ( a ) Sampling sites of bottom seawater. The displaced fault plane is shown as a box with thin hatched lines [4] . The dashed line and star indicate the volcanic front and hypocenter, respectively. The black bar at the top left denotes a 100-km scale bar. ( b ) The size of the coseismic slip during the earthquake estimated by land and seafloor geodesy [19] . The black bar at the top right denotes a 100-km scale bar. 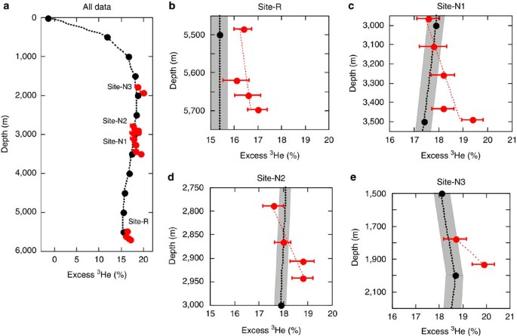Figure 2: Depth variations of helium isotope compositions in bottom seawater samples. The dotted curve shows the3He profile before the earthquake based on 69 measurements since 2007. Black and red solid circles indicate the average before the earthquake and after the earthquake, respectively. Bars represent one sigma error of samples after the earthquake. Shaded areas indicate the average values plus one sigma error before the earthquake. (a) Data at all sites. (b)3He profile at site R. (c)3He profile at site N1. (d)3He profile at site N2. (e)3He profile at site N3. Thin dotted red lines in (b) to (e) show the best fit lines obtained using the least squares method. Full size image Figure 2: Depth variations of helium isotope compositions in bottom seawater samples. The dotted curve shows the 3 He profile before the earthquake based on 69 measurements since 2007. Black and red solid circles indicate the average before the earthquake and after the earthquake, respectively. Bars represent one sigma error of samples after the earthquake. Shaded areas indicate the average values plus one sigma error before the earthquake. ( a ) Data at all sites. ( b ) 3 He profile at site R. ( c ) 3 He profile at site N1. ( d ) 3 He profile at site N2. ( e ) 3 He profile at site N3. Thin dotted red lines in ( b ) to ( e ) show the best fit lines obtained using the least squares method. Full size image Crustal fluids in the frontal arc A review of the available data shows that 3 He/ 4 He ratios in fluids are low in the frontal arc and high in the volcanic arc in subduction zones [11] . This spatial variation in 3 He/ 4 He is prominent in the Tohoku district (northeast region) of Japan (see Fig. 3a ) [12] , [13] , where crustal helium dominates, with a low 3 He/ 4 He ratio of ~0.3 Ra in deep-sea sediments and pore water in the trench region. 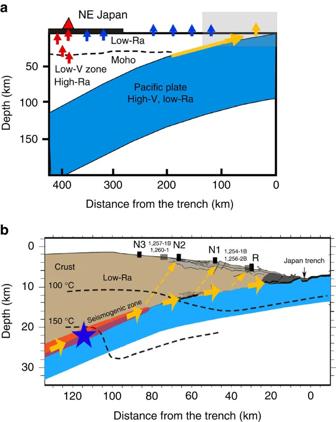Figure 3: Schematic cross-section of NE Japan and the Japan Trench. (a) A cross-section of the NE Japan arc with helium isotope signatures. Shaded region is enlarged inFig. 3b. V represents the velocity of seismic shear waves, and Ra represents the helium isotopic ratio relative to the atmosphere at 1.4 × 10−6. Red, yellow and blue arrows denote fluid emanation with helium isotopic ratios higher than 4 Ra, between 2 and 4 Ra, and lower than 2 Ra, respectively. The long yellow arrow indicates the mantle-derived fluid flow. (b) The thermal structures, including the seismogenic zone before the earthquake (red shape), estimated fluid flow (thick yellow arrows) and the hypocentre of the 11 March 2011, moment magnitude 9.0 Tohoku-Oki earthquake (blue star), are shown together with the bottom seawater and sediment sampling sites. Thin dashed yellow arrows indicate fluid transfer from the subsurface region to the sea bottom through a fault system. Light blue and brown areas are basaltic basement and Pleistocene accretionary prism, respectively. R, N1, N2, N3 indicate the sampling sites. This figure is modified from Kimuraet al.7 Analysis of the pore water in this work confirms the low values of 3 He/ 4 He ( Supplementary Table 3 and Methods). This finding is consistent with the advanced age of the descending Pacific plate, which is ~120 million years ago (Ma) [14] . Marine sediments might trap crustal helium degassed from the oceanic plate over geological time. Several papers reported helium isotope changes related to seismic activity [15] , [16] . Seismic activity would squeeze and expel such crustal helium trapped in sediments and slabs. This effect was observed during the Kobe earthquake in 1995 (ref. 17 ) when the 3 He/ 4 He ratio of the groundwater decreased in the city of Nishinomiya, which is close to Kobe, immediately after the earthquake, and the 4 He/ 20 Ne ratio increased markedly, suggesting the input of crustal helium into the aquifer because of the earthquake. If the Tohoku-Oki earthquake forced sediments to expel pore fluids, the 3 He/ 4 He ratio of the bottom seawater should decrease. However, this was not the case. Elevated 3 He/ 4 He ratios were found in the bottom seawater of the frontal arc region 1 month after the earthquake. Figure 3: Schematic cross-section of NE Japan and the Japan Trench. ( a ) A cross-section of the NE Japan arc with helium isotope signatures. Shaded region is enlarged in Fig. 3b . V represents the velocity of seismic shear waves, and Ra represents the helium isotopic ratio relative to the atmosphere at 1.4 × 10 −6 . Red, yellow and blue arrows denote fluid emanation with helium isotopic ratios higher than 4 Ra, between 2 and 4 Ra, and lower than 2 Ra, respectively. The long yellow arrow indicates the mantle-derived fluid flow. ( b ) The thermal structures, including the seismogenic zone before the earthquake (red shape), estimated fluid flow (thick yellow arrows) and the hypocentre of the 11 March 2011, moment magnitude 9.0 Tohoku-Oki earthquake (blue star), are shown together with the bottom seawater and sediment sampling sites. Thin dashed yellow arrows indicate fluid transfer from the subsurface region to the sea bottom through a fault system. Light blue and brown areas are basaltic basement and Pleistocene accretionary prism, respectively. R, N1, N2, N3 indicate the sampling sites. This figure is modified from Kimura et al. [7] Full size image Origin of high helium-3 The plot of 20 Ne/ 4 He and 3 He/ 4 He ratios shows two end members: one with low 20 Ne/ 4 He and high 3 He/ 4 He and the other with high 20 Ne/ 4 He and low 3 He/ 4 He ( Supplementary Fig. 4 ). The latter falls with the value of the northwest Pacific bottom water. The end member with high 3 He/ 4 He has an Ra of 2.4±0.6. This value is markedly higher than those of the atmosphere and pore water in the hypocentre region (0.68–0.71 Ra) and trench region (0.15–0.77 Ra) [13] . It may be argued that the excess 3 He was derived from tritiogenic 3 He from the Fukushima nuclear reactor; however, we rejected this possibility because the 3 He would have come from the surface, and the observed depth profile shows a higher 3 He in deeper samples ( Fig. 2b–e ). As previously mentioned, the oceanic crust is old and is expected to contain radiogenic [14] isotopes. Therefore, the crust is not the source of the elevated 3 He/ 4 He ratios. Cosmic dust in sediments with a high 3 He/ 4 He ratio might contribute to the high 3 He (ref. 18 ); however, we measured the solid sediment and found that the ratio is low, with values of 0.1–0.8 Ra (see Supplementary Table 2 ). Below 2,500 m of seawater, excess 3 He would decrease with depth, which is a positive inclination in the depth profile ( Fig. 2a and Supplementary Fig. 2 ). If the tsunami following the M9.0 earthquake triggered vertical mixing of deep seawater and/or a mass movement of water, the excess 3 He may have increased in deeper regions. However, the mixing cannot produce the negative inclination that was observed after the earthquake ( Fig. 2b–e ), even if the mixing had homogenized the excess 3 He and made an infinite inclination. In addition, there are no significant changes in the depth profiles of temperature and salinity observed by the CTD (conductivity, temperature, depth) rosette before and after the earthquake. Finally, there is a positive relationship between the excess 3 He and the methane contents in these samples ( Supplementary Fig. 5 ), which suggests that a percentage of methane may be derived along with the 3 He. The vertical mixing of seawater and/or mass movement of water cannot produce such a correlation because both were derived below the seafloor. Consequently, it is difficult to find the source of the excess 3 He within the water and from the atmosphere. The most probable origin is mantle fluid from the mantle wedge that was released into the trench region through the boundary of the descending oceanic and over-riding plates. The mantle fluid hypothesis is supported by the displaced fault plane of 440 × 220 km (ref. 4 ) during the Tohoku-Oki earthquake, of which the deepest portion reaches the mantle depth ( Fig. 1a ). It is worth noting that the slip of the M9.0 earthquake is anomalously large and exceeds 50 m in regions close to several bottom-water sampling sites [19] . The coseismic slip likely created a dilation through which fluid flowed from the mantle depth. Geophysical and geological studies [6] , [7] , [8] have suggested the existence of highly pressurized fluids along the plate interface. Such fluids might move along the plate interface from the upper mantle to the trench ( Fig. 3a ) or transfer from the subsurface region to the sea bottom through a fault system in the trench ( Fig. 3b ). Abundant evidence exists for the emanation of mantle helium traversing the crust along a strike slip, such as what is found in the San Andreas fault [20] , the Anatolian fault in Turkey [21] and the major normal and oblique normal faults in the Basin and Range [22] . However, these data are in steady state with a continuous emission of mantle helium. Our observations represent the first findings of a non-steady-state, catastrophic emanation of mantle helium that was likely induced by the M9.0 earthquake. The distance from the nose of the mantle wedge to the trench surface is ~150 km. As measurements were taken 35 days after the M9.0 earthquake, the estimated fluid flow velocity was greater than 4 km per day, which is 2 orders of magnitude higher than the fluid migration estimated by a numerical model of the pressure solitary wave propagation in the Nankai wedge of SW Japan [23] . The fluid flow velocity was estimated during the 1986 eruption of the Oshima volcano in Japan [24] . A time lag between the eruption and enhancement of the 3 He/ 4 He ratios in the steam located 3 km from the central crater implied a velocity greater than 50 m per day. The value is much smaller than the value obtained in this study. During volcanism of the Miyakejima island in 2000, fluid migration was suggested by seismic activity [25] . The estimated velocity is extremely high, with a value of 5–10 km per day, which is equivalent to our results. For the Tohoku-Oki earthquake, a slow-slip propagation accompanying foreshock activity was observed in the region of the main rupture before the M9.0 earthquake [26] . If the slip propagation is related to the movement of fluids, then the velocity of 2–10 km per day is similar to what was calculated for the main rupture in this study, even though the direction of the slow-slip propagation is along the trench axis, which is different from the direction across the arc of the hypothetical mantle fluid flow. Slow-slip events have been detected on fault patches with extremely low frictional strength [27] . The weakness is attributable to increased pore-fluid pressure and may be linked to the release of fluids from the descending plate to the mantle [28] ( Fig. 3 ). The slow-slip event before the main earthquake suggests that the mantle fluid may have already been in the seismogenic zone, implying a much shorter flow path to reach the sea floor. The existence of fluids may decrease the effective normal stress in the region, thereby triggering the M9.0 earthquake. If the 3 He-rich fluid was already in the epicentre, the distance from the main shock region to the trench surface is reduced to 30–40 km and the velocity of the fluid is ~1 km per day, suggesting that the calculated velocity has an error of a factor of 4. Elevated pore-fluid pressure and the rupture of fault plane likely enhanced the rapid flow ( Fig. 3 ). It is possible to calculate the regional 3 He flux from the mantle to the ocean during this event based on the gradient of excess 3 He (2–3%) at specific depths and a simple steady-state diffusion model [29] , [30] , assuming that the vertical advection and horizontal diffusion are negligible. The 4 He/ 20 Ne ratios are constant with depth within the analytical error at sites N1, N3 and R, whereas the ratios increase slightly with depth at site N2 ( Supplementary Fig. 6 ). Assuming that neon has a constant concentration of 1.86 × 10 −7 ccSTP g H20 −1 in seawater [9] , the observed 4 He/ 20 Ne ratios produce 3 He gradients of 1.2 × 10 −20 ccSTP g −1 cm −1 at site R, 1.5 × 10 −20 ccSTP g −1 cm −1 at site N1, 5.0 × 10 −20 ccSTP g −1 cm −1 at site N2 and 4.4 × 10 −20 ccSTP g −1 cm −1 at the site N3 ( Supplementary Table 4 ). Assuming that the vertical eddy diffusivity is constant with the value of 1.0 cm 2 s −1 (refs 29 , 30 ), the estimated 3 He fluxes are calculated to be 0.3±0.4 atoms cm −2 s −1 at site R, 0.4±0.2 atoms cm −2 s −1 at site N1, 1.4±0.6 atoms cm −2 s −1 at site N2 and 1.2 atoms cm −2 s −1 at site N3, where the errors are one sigma. For the site N3, it is difficult to calculate the error because of the two data points. These 3 He fluxes are the first data obtained in a trench region with significantly large values, comparable to the ~1 atom cm −2 s −1 value observed in the back-arc basin hydrothermal system in the Mid-Okinawa Trough [31] . It is informative to convert these 3 He fluxes to primordial heat fluxes based on the global relationship between the two [13] , [32] fluxes. Estimated heat fluxes in the area are 0.6–2.5 mW m −2 , which is markedly less than the terrestrial heat flow values of 22–32 mW m −2 observed in the Japan Trench [33] . Helium may diffuse faster and farther than heat, which is well documented around the Ontake Volcano, Japan [34] . At the site, excess 3 He was observed 25 km away from the central cone, and there is no heat anomaly at 15 km; therefore, it is difficult to detect a heat anomaly related to the discharge of fluids during the M9.0 earthquake. However, an influx of 13 C-enriched methane was observed in the same samples along with the light transmission anomaly and a variation of prokaryotic biomass [35] . CH 4 / 3 He ratios can be calculated by the excess 3 He relative to the steady-state 3 He depth profile of the Pacific Ocean water before the earthquake ( Fig. 2 ) and the CH 4 content [35] . The CH 4 / 3 He ratios vary from 5.5 × 10 7 to 2.4 × 10 9 ( Supplementary Table 4 ), which is greater than the 2 × 10 6 –1 × 10 7 ratio from hydrothermal fluids in the East Pacific Rise (EPR) [36] . The reported δ 13 C values (−45 to −87‰) of samples collected shortly after the M9.0 earthquake ( Supplementary Table 4 ) are much lower than the values expected in the mantle and the EPR, approximately −23‰ (ref. 37 ). Therefore, the methane cannot simply be derived from the upper mantle. The δ 13 C value of −80‰ at site R is in agreement with the biogenic methane of the shallow sediment in the region where the 3 He flux is relatively small. In contrast, 13 C-rich methane with δ 13 C values of approximately −60‰ was recorded at sites N1, N2 and N3. The 3 He/ 4 He ratio of the non-atmospheric end member was estimated to be 2.4±0.6 Ra. The data suggest a 30% contribution from the upper mantle helium of 8 Ra and crustal helium of 0.3 Ra. Conversely, a binary mixing of two components, EPR-type methane with δ 13 C=−23‰ and CH 4 / 3 He=6 × 10 6 and crustal methane with δ 13 C=−60‰ and CH 4 / 3 He=1 × 10 10 , may be applicable to the samples at sites N1, N2 and N3 ( Supplementary Fig. 7 ). The estimated EPR-type methane fractions vary from 0.2 to 9.0%, with an average of 2.5%. This result suggests that pre-fluids from the seismogenic zone along the plate interface likely contained a small portion of abiogenic methane. In contrast to the 3 He/ 4 He ratios in deep seawater in June 2011 ( Supplementary Fig. 3 ), bottom samples at shallow depths (sites 2, 3 and DT99) do not show excess 3 He relative to the pre-earthquake values, which suggests that emanation of the mantle helium had ceased and that the anomaly was dissipated by diffusion in a horizontal direction ( Supplementary Fig. 8 and Methods). Conversely, excess 3 He was found in deeper samples (sites 5, 7 and 8) 3 months after the M9.0 earthquake, which suggests either a continuing emanation of mantle helium or a slow horizontal dissipation in a deep narrow basin-like trench structure. Finally, a helium anomaly was not found in pore-water samples of a coseismic slip zone in August 2011, supporting the conclusion that the helium isotope signature is generally crustal in the frontal arc region of NE Japan and that the emanation of mantle helium is in a non-steady-state influx. In conclusion, elevated 3 He/ 4 He ratios were observed in bottom seawater samples in the main shock region of the 2011 M9.0 Tohoku-Oki earthquake. The anomaly might derive from the mantle through the plate interface, most likely induced by over-pressured pore fluids and methane. This is the first reported finding of mantle-derived helium released through the plate interface in subduction zones. Sampling and analysis To study the coseismic and post-seismic impacts on the geochemical state of the mainshock region of the 2011 M9.0 Tohoku-Oki earthquake, we collected near-bottom seawater samples from several depths at four seafloor sites ( Fig. 1 ; sites R (38°12.5′N, 143°47.2′E), N1 (38°10.6′N, 143°33.0′E), N2 (38°8.7′N, 143°19.0′E) and N3 (38°6.8′N, 143°5.0′E)) on 15 April 2011 by CTD–CMS (Carousel Multi Sampling System) hydrocasts during the MR11-03 cruise of R/V Mirai . A second set of bottom seawater samples was taken at six sites ( Fig. 1a ; stations 2 (38°9.7′N, 143°26.4′E), 3 (38°8.7′N, 143°19.0′E), 5 (38°12.6′N, 143°47.1′E), 7 (37°39.4′N, 143°40.6′E), 8 (37°40.7′N, 143°33.7′E) and DT99 (37°44.4′N, 143°17.0′E)) on 16 June 2011 during the YK11-E04 cruise of R/V Yokosuka . Deep-sea sediment and pore-water samples were collected at four sites (1254-1B (37°45′N, 143°17′E), 1256-2B (39°7′N, 143°53′E), 1257-1B (37°45′N, 143°17′E) and 1260-1 (37°45′N, 143°17′E)) during the YK11-E06 cruise of R/V Yokosuka ( Fig. 3b ). In the laboratory, helium and neon were extracted from the seawater and pore water in the sediment and purified using hot Ti-getters and charcoal traps held at 77 K. The 4 He/ 20 Ne ratios were measured using a quadrupole mass spectrometer. The helium was then separated from the neon by a charcoal trap held at 40 K. The 3 He/ 4 He ratios were measured using a high-precision mass spectrometer (Helix SFT; GV Instruments Ltd.) and calibrated against our in-house standard (HESJ) [38] . Experimental errors of 3 He/ 4 He and 4 He/ 20 Ne ratios were ~0.4 and 3%, respectively, at one sigma. We also measured the 3 He/ 4 He and 4 He/ 20 Ne ratios of sediment samples by a pyrolysis experiment using a vacuum tantalum furnace. The errors are larger than those of seawater samples because of smaller amounts of noble gas. Pre-earthquake 3 He profile Before the M9.0 earthquake, we collected 69 seawater samples northeast of Sendai in the northwestern Pacific ( Supplementary Fig. 1 ) from May 2007 to June 2010 by several cruises of the R/Vs Hakuho and Tansei . The sampling dates and locations are listed in Supplementary Table 5 . The sites are located between 100 and 200 km from the hypocentre and within the displaced fault plane (440 × 220 km), except for site KH08-3-C023. Most of the sites are situated in a coseismic slip zone ( Fig. 1b ). Depth profiles for all excess 3 He data are shown in Supplementary Fig. 2 . The dotted line is obtained by a weighted mean average of data at the same depth. Numerical data are listed in Supplementary Table 6 . The estimated error of the depth between 2,000 and 5,000 m is significantly small (~0.3%). Therefore, the ‘pre-earthquake 3 He profile’ may represent the helium isotope signature of deep seawater in the region before the M9.0 earthquake. A maximum 3 He excess was observed at a depth of 2,000–2,500 m ( Supplementary Fig. 2 ), which is consistent with the anomaly in the East Pacific Rise at 15°S (ref. 39 ) and apparently deeper than that of the Okinawa Trough [40] . Therefore, the excess 3 He is derived from long distance transportation by the abyssal current at ~10,000 km (ref. 10 ). This movement may homogenize the 3 He/ 4 He signatures at the same depth for several hundred kilometres in a horizontal direction, which would assure the robustness of the normal 3 He profile in the trench region before the earthquake. Source of deep-sea sediment in a coseismic slip region The soft sediment samples at the seafloor basement were collected in a region of a coseismic slip zone by the HOV Shinkai6500 . The sediments are composed of dark-olive silt and grey sandy silt intercalated with thin sand layers, implying a turbidite signature. The hinterland provenance of the sediment may be the Kitakami Mountain, a non-volcanic fore-arc region in the Tohoku district. The basement is composed of Mesozoic and Paleozoic layers, and the 3 He/ 4 He ratio may have a crustal signature that is significantly lower than 1 Ra. The variation of helium isotopes in the sediments (0.11–0.79 Ra) is most likely attributable to the mixing of the crustal helium and cosmic dust helium of ~300 Ra (ref. 18 ). Temporal variation of excess 3 He in deep seawater We have examined helium isotopes of deep seawater samples collected northeast of Sendai in the northwest Pacific before and after the M9.0 earthquake. Temporal variations of excess 3 He at several depths are plotted against the sampling data in Supplementary Fig. 8 . From May 2007 to June 2010, the excess 3 He was generally constant. One month after the M9.0 earthquake, all depth data showed a significant increase in excess 3 He. The values then returned to the normal 3 He profile, except for the deepest samples (5,000–6,000 m). This result may suggest that the emanation of the mantle helium was catastrophic and ceased at the shallower sites in June 2011, which is confirmed by the low 3 He/ 4 He ratios ( Supplementary Table 3 ) in the pore-water samples collected in August 2011 and consistent with the idea that 3 He/ 4 He ratios of fluid samples are low in the frontal arc [11] , [12] . We also statistically examined the 3 He anomaly in two data sets: the average of seawater helium isotopes based on four to five measurements before the M9.0 earthquake ( Supplementary Fig. 8 ) and the helium isotopes measured ~1 month after the M9.0 event. The former has an error of average from the analysis of the four to five measurements (error_a), and the latter is from the helium isotope measurement (error_s). The combined errors should be calculated in quadrature by the sqrt (error_a 2 +error_s 2 ). For example, we consider the data set of depth=3,000 m ( Supplementary Tables 1 and 6 ). The average of excess 3 He before the M9.0 earthquake is 17.9±0.2% at 1 sigma. Measurement after the event shows an average of excess 3 He of 18.8±0.4% at 1 sigma. In this case, the combined error becomes 0.45% at 1 sigma. The 2 sigma value of the combined error is 0.9%, which agrees with the difference of the average (17.9%) and the measurement (18.8%). This result suggests that the anomaly exists at 3,000 m at a 95% confidential level. For the 2,000-m data set, the anomaly is valid again at the 95% level. For the 3,500 m and 5,000–6,000 m data sets, the differences are larger than the 2-sigma value, suggesting that the anomaly is statistically valid. Therefore, all four depths ( Supplementary Fig. 8 ) show robust evidence of a helium-3 anomaly in the temporal variation. How to cite this article : Sano, Y. et al. Helium anomalies suggest a fluid pathway from mantle to trench during the 2011 Tohoku-Oki earthquake. Nat. Commun. 5:3084 doi: 10.1038/ncomms4084 (2014).